Sulfisoxazole does not inhibit the secretion of small extracellular vesicles 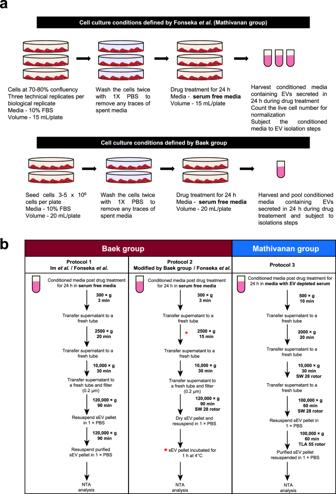Fig. 1: Schematic representation of cell culture, drug treatment and sEV isolation by two groups. aSchematic representation of cell culture and drug treatment approaches. The cells were seeded and allowed to grow to 70–80% confluency in media supplemented with FCS. Upon attaining desired confluency, cells were washed with 1× PBS and subjected to drug treatment for 24 h in serum-free media. At treatment endpoint, conditioned media was harvested and subjected to sEV isolation. Live cell number was determined to normalise particles released to cell number. Similarly, Baek group seeded cells in a pre-defined range and treated them with drug in serum-free media.bProtocol 1, schematic flow diagram depicting the methodology of sEV isolation and analyses as defined by Baek group in the initial publication (Im et al.13) and followed by Fonseka et al. (this study). Protocol 2, schematic flow diagram depicts the methodology of sEV isolation and analyses as reported by Baek group when approached. The variations in the methodology from the original manuscript (Im et al.) is marked (*). Protocol 2 was also adapted by Fonseka et al. to include the variations (*) suggested by Baek group. Protocol 3, standardized and optimized method of sEV isolation in EV depleted serum used in Mathivanan laboratory was also used to collect sEVs post treatment with SFX. 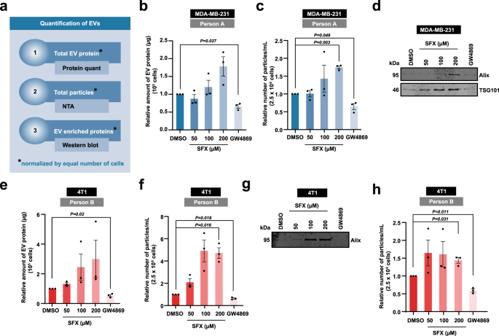Fig. 2: Quantification of EVs released by cells with or without SFX and GW4869. aSchematic of EV quantification by three different methods. Firstly, the total EV protein amount was quantified and normalised to equal number of live cells. Secondly, nanoparticle tracking analysis (NTA) was performed to quantify the total number of particles normalised to equal number of live cells. Lastly, Western blot analysis of EV samples obtained from equal number of live cells was performed for EV enriched proteins.bRelative amount of EV protein normalised to 105MDA-MB-231 cells is shown.cRelative number of particles normalised to 2.5 × 106MDA-MB-231 cells is depicted.dWestern blot analysis of EV enriched proteins Alix and TSG101 in EV samples obtained from 15 × 106MDA-MB-231 cells. Representative image shown,n=3biologically independent experiments.eRelative amount of EV protein normalised to 1054T1 cells is shown.fRelative number of particles normalised to 2.5 × 1064T1 cells is depicted.gWestern blot analysis of EV enriched proteins Alix in EV samples obtained from 15 × 1064T1 cells. Representative image shown,n=3biologically independent experiments.hRelative number of particles normalised to 2.5 × 1064T1 cells is depicted. All data are represented as mean ± s.e.m.n= 3 biologically independent experiments, statistical significance was determined by paired two-tailedt-test. EVs were isolated by protocol 1 (b–g) and 2 (h). Full uncropped images for western blotting is provided in Supplementary Fig.1. Cell culture Human breast cancer cell line MDA-MB-231 was obtained from ATCC and murine breast cancer cell line 4T1 was gifted by Dr. Belinda Parker (La Trobe University). Cells were cultured at 37 °C, 5% CO 2 , and 95% humidity in the presence of 10% fetal calf serum (FCS - Assay Matrix #ASFBS) and 100 Unit/mL penicillin-streptomycin (GIBCO, Life Technologies). Alpha minimum essential medium (GIBCO, Life Technologies) was used for growing 4T1 cells whereas MDA-MB-231 cells were grown in Dulbecco’s modified Eagle’s medium (GIBCO, Life Technologies). Isolation of EVs For protocol 1 (Fig. 1 ), EVs were isolated by exactly following the method reported by Im et al. [13] . Briefly, 4T1 and MDM-MB-231 cells were cultured until 80% confluence and were washed with 1× PBS and incubated in vehicle or SFX (Merck #31739) for 24 h in serum-free media. The conditioned media was then subjected to differential centrifugation (300 × g for 3 min, 2500 × g for 20 min and 10,000 × g for 30 min). Next, the supernatant was filtered using 0.2 μm filter followed by a centrifugation at 120,000 × g for 90 min. The EV pellet was then resuspended in PBS and subjected to another centrifugation at 120,000 × g for 90 min. The obtained EV pellet was then resuspended in PBS for further experiments. For protocol 2 (Fig. 1 ), EVs were isolated with slight modifications from protocol 1 (differential centrifugation 2500 × g for 15 min and sEV incubated for 1 h at 4 °C). The modifications in protocol 2 as compared to protocol 1 is denoted with * in Fig. 1b . For protocol 3, EVs were isolated by Mathivanan laboratory methods as described previously [15] . Briefly, conditioned media was collected and centrifuged at 500 × g for 10 min to remove cell debris followed by 2000 × g for 20 min at 4 °C. The supernatant was subjected to centrifugation at 10,000 × g for 30 min at 4 °C to remove large extracellular vesicles. The supernatant was then subjected to ultracentrifugation at 100,000 × g (SW28 rotor, Beckman) for 1 h at 4 °C. This step was repeated to wash the pellet with 1× PBS to collect sEVs for further analysis. Protein quantification Equal volumes of EV samples were suspended in sodium dodecyl sulphate (SDS) buffer (8% w/v SDS, 10% v/v glycerol, and 0.4% v/v bromophenol blue, 200 mM Tris‐hydrochloride (Tris‐HCl), pH 6.8) with 100 m M dithiothreitol (DTT)). The protein samples were then heated at 92 °C for 2 min. The samples were resolved in SDS-PAGE at 150 V for 1 h followed by overnight SYPRO ruby staining according to manufactures instructions (Invitrogen™- S12000). Gels were then scanned using Typhoon™ FLA 9500 (GE Healthcare Life Sciences). Densitometric analysis was performed through ImageQuant™ to determine the protein concentration relative to a BenchMark™ Protein Ladder (Invitrogen). The obtained protein amount was then normalised to equal number of cells (1 × 10 5 ). Nanoparticle tracking analysis (NTA) EVs were analysed using NanoSight N300 (Malvern Instruments, Malvern, UK). The samples were monitored with the laser Monochromatic laser beam at 405 nm. EV sample volume was normalised to equal number of MDA-MB-231 and 4T1 (2.5 × 10 6 ) cells. Three videos of 30 s each were taken for each sample (replicate). All the parameters and settings were maintained to be constant throughout the experiment (camera level at 12, detection threshold at 5 and syringe pump speed at 50 and temperature at 25 °C). Results obtained were analysed using NTA software 3.0 (ATA Scientific). Western blotting analysis EV sample were normalised to equal number of cells (15 × 10 6 ) before subjecting to lysis in SDS sample buffer. The protein samples were then resolved in SDS-PAGE at 150 V for 1 h. The resolved proteins were transferred onto a nitrocellulose membrane (Thermo Scientific™) using a wet transfer system at 25 V for 2.5 h in transfer buffer (11.5 mM Tris, 95 mM Glycine, 20% (v/v) Methanol). The membrane was blocked using 10% (w/v) skim milk in TTBS (100 mM Tris-HCl pH 7.5, 150 mM NaCl, 0.05% (v/v) Tween 20) for 1 h at room temperature. Next, the membrane was washed three times (10 min each) with TTBS before incubating in primary antibodies Alix (Cell Signaling Technology #2171S) and TSG101 (BD Transduction Laboratories #612696) over night at 4 °C (1:1000 dilution). Same wash cycle was applied following incubation with secondary antibody (IRDye 800CW secondary anti-mouse - LI-COR ® ) at room temperature for 1 h (1:10,000 dilution). Membrane was then washed three times with TTBS prior to visualisation using Odyssey® CLx (LI-COR ® ). Reporting summary Further information on research design is available in the Nature Research Reporting Summary linked to this article.